Disease mutations in the ryanodine receptor N-terminal region couple to a mobile intersubunit interface Ryanodine receptors are large channels that release Ca 2+ from the endoplasmic and sarcoplasmic reticulum. Hundreds of RyR mutations can cause cardiac and skeletal muscle disorders, yet detailed mechanisms explaining their effects have been lacking. Here we compare pseudo-atomic models and propose that channel opening coincides with widening of a cytoplasmic vestibule formed by the N-terminal region, thus altering an interface targeted by 20 disease mutations. We solve crystal structures of several disease mutants that affect intrasubunit domain–domain interfaces. Mutations affecting intrasubunit ionic pairs alter relative domain orientations, and thus couple to surrounding interfaces. Buried disease mutations cause structural changes that also connect to the intersubunit contact area. These results suggest that the intersubunit contact region between N-terminal domains is a prime target for disease mutations, direct or indirect, and we present a model whereby ryanodine receptors and inositol-1,4,5-trisphosphate receptors are activated by altering domain arrangements in the N-terminal region. Ryanodine receptors (RyRs) are ion channels that govern the release of Ca 2+ from the endoplasmic or sarcoplasmic reticulum [1] . They are involved in many physiological events, including excitation–contraction coupling. In mammalian organisms, three different isoforms have been identified (RyR1-3) [2] , [3] , [4] . RyR1 is mainly found in skeletal muscle, whereas RyR2 is the isoform that predominates in cardiac myocytes. RyR mutations can result in severe disease phenotypes. More than 300 have been identified in RyR1, associated with malignant hyperthermia (MH) [5] , central core disease and related conditions [6] . In the cardiac isoform, more than 150 mutations have been linked to catecholaminergic polymorphic ventricular tachycardia [7] , arrhythmogenic right ventricular dysplasia type 2 and idiopathic ventricular fibrillation [8] . Many mutations cluster in three distinct ‘hot spots’ within the sequence, but several others, especially for RyR1, are increasingly found outside of these clusters ( Supplementary Fig. S1 ). The primary trigger for RyR opening is Ca 2+ , the same ion it permeates. RyRs can be activated by either cytoplasmic or luminal Ca 2+ ions [9] , [10] , but higher cytoplasmic Ca 2+ concentrations can inhibit RyRs [11] . In skeletal muscle, RyR1 can also be triggered to open through conformational changes in the L-type calcium channel Ca V 1.1, which is thought to interact directly with RyR1 (ref. 12 ). In addition, a host of regulatory proteins and small molecule ligands can alter the sensitivity to these primary triggers. The precise mechanisms by which Ca 2+ or Ca V 1.1 alter channel gating are still unknown. Several high- and low-resolution studies have shed light on the RyR structure [13] . Cryo-electron microscopy (cryoEM) studies depict a mushroom-shaped structure with the stem forming the transmembrane region, and the cap located in the cytoplasm [11] , [12] . A study comparing the open and closed states suggests that channel opening is the result of inner transmembrane helices that bend, in agreement with high-resolution studies on other ion channels [14] . However, helix bending in RyRs is still a contentious issue [15] . Channel opening also coincides with many movements in the cytoplasmic area, showing that RyRs are bona fide allosteric proteins. As a result, RyR-interaction partners that bind far away from the pore region can influence channel opening. For example, any partner that preferentially stabilizes the open state can facilitate channel opening. The overall open probability is thus the result of the integrated effect of ligands with positive and negative input. Similarly, any mutation that selectively affects one of the states may facilitate or inhibit channel opening. Several crystallographic studies have shed light on RyR domains [16] , [17] , [18] , [19] , [20] , [21] . The N-terminal region (RyR1 residues 1–532), containing the bulk of the proposed N-terminal disease hot spot, is built up by three domains (‘A’, ‘B’ and ‘C’) ( Supplementary Fig. S1 ) and forms a cytoplasmic vestibule [16] . This position was recently confirmed via a cryoEM reconstruction, whereby green fluorescent protein was inserted in RyR2 domain B [22] . For simplicity, we refer to the three domains together as the N-terminal disease hot spot. In the related inositol-1,4,5-trisphosphate receptor (IP 3 R), the corresponding region forms the binding site for IP 3 , which triggers channel opening [23] , [24] . However, a direct functional role for the RyR N-terminal domains is unknown. Most mutations studied so far seem to confer a gain-of-function phenotype, whereby channel opening is facilitated [1] . However, some mutations associated with central core disease and idiopathic ventricular fibrillation, mostly located in the transmembrane area, can confer a loss-of-function [25] , [26] . How can N-terminal disease mutations, located >100 Å away from the transmembrane inner helices, facilitate channel opening? Most of them are found at domain–domain interfaces, suggesting that perhaps some or all of these interfaces undergo changes during channel opening, and that disease mutations directly interfere with such events. Here we compare pseudo-atomic models of the N-terminal area in the open and closed states, and look at crystal structures of disease mutations that affect domain–domain interactions. We present a model whereby neighbouring N-terminal hot spots interact through an interface that is disrupted upon channel opening. Pseudo-atomic models of the N-terminal disease hot spot The opening of RyRs is allosterically coupled to the cytoplasmic cap, which undergoes large conformational changes [14] , [27] , [28] , [29] . This includes movements in the central rim, a region surrounding the four-fold symmetry axis on the cytoplasmic face, where the N-terminal disease hot spot was found to be located [16] , [22] . We therefore docked the crystal structure of the RyR1 N-terminal domains (RyR1ABC) in the open- and closed-state cryoEM maps of RyR1, previously compared in a systematic study at 10.2 Å [14] . Consistent with previous results in three other RyR1 cryoEM maps [16] , RyR1ABC docks around the four-fold symmetry axis with a high docking contrast, whereby the top solution clearly stands out from the next solutions down the ranking ( Fig. 1a ). As it is possible that the individual domains A, B and C also undergo relative movements during channel opening, we further refined their positions in both maps by allowing a flexible fit of each individual domain. 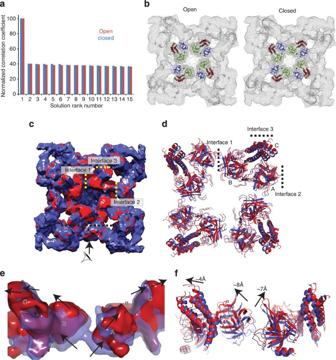Figure 1: Pseudo-atomic models of RyR1ABC in open and closed RyR1. (a) Docking contrasts for RyR1ABC docking, before refinement of the individual domain positions, in the open (red) and closed states (blue), showing the Laplacian-filtered cross-correlation coefficients for the top 15 unique positions. The correlation coefficients are normalized to the highest score. (b) Positions of RyR1ABC (Protein Data Bank (PDB) ID: 2XOA) docked in the open (left, EMDB 1607) and closed (right, EMDB 1606) RyR1 cryoEM maps. Different colours indicate the individual domains (A: blue, B: green and C: red). (c,d) Top view (cytoplasmic face) of a superposition of the entire cryo-EM maps and the docked RyR1ABC domains after refinement of the individual domain positions in closed (blue) and open (red) RyR1. The arrow and black dotted line incindicate a cross-section used for the side view ine. (e,f) Side view of the cryoEM maps and the docked RyR1ABC domains. The portion of the maps shown is based on segmentation through Segger, as a plug-in for Chimera54. The docked positions are also shown inSupplementary Movies 1 and 2. Figure 1b shows their final refined positions. A direct superposition of these pseudo-atomic models shows that there are substantial shifts up to 8 Å ( Fig. 1c–f , Supplementary Movies 1,2 ). The major rearrangement in the models can be described as ‘tilting’, whereby all domains move upward and outward, as if pivoting around a hinge outside the hot spot. Figure 1: Pseudo-atomic models of RyR1ABC in open and closed RyR1. ( a ) Docking contrasts for RyR1ABC docking, before refinement of the individual domain positions, in the open (red) and closed states (blue), showing the Laplacian-filtered cross-correlation coefficients for the top 15 unique positions. The correlation coefficients are normalized to the highest score. ( b ) Positions of RyR1ABC (Protein Data Bank (PDB) ID: 2XOA) docked in the open (left, EMDB 1607) and closed (right, EMDB 1606) RyR1 cryoEM maps. Different colours indicate the individual domains (A: blue, B: green and C: red). ( c , d ) Top view (cytoplasmic face) of a superposition of the entire cryo-EM maps and the docked RyR1ABC domains after refinement of the individual domain positions in closed (blue) and open (red) RyR1. The arrow and black dotted line in c indicate a cross-section used for the side view in e . ( e , f ) Side view of the cryoEM maps and the docked RyR1ABC domains. The portion of the maps shown is based on segmentation through Segger, as a plug-in for Chimera [54] . The docked positions are also shown in Supplementary Movies 1 and 2 . Full size image These overall shifts are also visible when comparing the corresponding density in the open- and closed-state cryoEM maps ( Fig. 1c ) [14] . A key observation is that the changes are concerted: where density is systematically disappearing ‘below’ the domains, extra density appears ‘above’ ( Fig. 1e ). Such concerted movements are highly improbable as a result of poor resolution or noise in the maps, as this would only cause random scatter in both directions. Although these pseudo-atomic models do not allow a detailed description of interactions across subunits, they imply that domains A and B of neighbouring subunits are juxtaposed, likely forming interactions in the closed state (‘interface 1’). However, in the open-state model, the intersubunit gap is extended by ~7 Å, a distance that is undoubtedly large enough to break or alter many interactions ( Fig. 2a ). Incidentally, the largest concentration of disease mutations in the N-terminal region is found facing the intersubunit boundary (20 for RyR1 and RyR2 combined). The bulk of the mutations are clustered in only three loops that are juxtaposed. One of these loops is located in domain A (connecting β strands 8 and 9), and was previously found to contain a dense cluster of mutations [17] , [18] . The two other loops reside in domain B and are inherently flexible in the absence of their binding partner ( Fig. 2a , red dotted lines). How could these mutations affect channel opening? Mutations in the β8-β9 loop were previously found not to cause any structural or stability differences [17] , [18] . This implies that the only way they can have an impact is by being directly involved in a functional interface, and we propose that they form part of intersubunit interactions that are disrupted upon channel opening. Any mutation that weakens these interactions will lower the energetic barrier to open the channel, and thus facilitate channel opening. 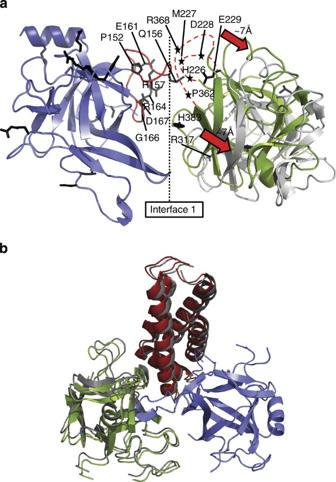Figure 2: Relative positions between and within N-terminal disease hot spots. (a) Superposition of domain A (blue) in the open- and closed-state models, showing the relative position of domain B in a neighbouring subunit (closed: green and open: grey). Disease mutations are shown as black sticks. Select mutations in three juxtaposed loops are labelled. The β8–β9 loop in domain A is shown in red. Two flexible loops in domain B that contain multiple disease mutations are shown as red dotted lines, with disease mutations indicated by black asterisks. This interface is subject to a total of 20 disease mutations: P152S*, Q156K, R157Q*, E161G, R164C, R164L, R164Q*, G166R, D167N, D167G, H226R*, M227K, D228V, E229K*, R317L, R317W*, P362M*, R368L, R368Q and H383N, where asterisks indicate mutations found in RyR2 (all in rabbit RyR1 residue numbering). (b) Superposition of the closed (colours) and open (grey) RyR1ABC models, based on domain A (blue), indicating the relative positions of domains B (green) and C (red). These conformational changes are too small to be interpreted at the resolution of the cryoEM maps, so channel opening does not seem to induce major conformational rearrangements within each hot spot. Figure 2: Relative positions between and within N-terminal disease hot spots. ( a ) Superposition of domain A (blue) in the open- and closed-state models, showing the relative position of domain B in a neighbouring subunit (closed: green and open: grey). Disease mutations are shown as black sticks. Select mutations in three juxtaposed loops are labelled. The β8–β9 loop in domain A is shown in red. Two flexible loops in domain B that contain multiple disease mutations are shown as red dotted lines, with disease mutations indicated by black asterisks. This interface is subject to a total of 20 disease mutations: P152S*, Q156K, R157Q*, E161G, R164C, R164L, R164Q*, G166R, D167N, D167G, H226R*, M227K, D228V, E229K*, R317L, R317W*, P362M*, R368L, R368Q and H383N, where asterisks indicate mutations found in RyR2 (all in rabbit RyR1 residue numbering). ( b ) Superposition of the closed (colours) and open (grey) RyR1ABC models, based on domain A (blue), indicating the relative positions of domains B (green) and C (red). These conformational changes are too small to be interpreted at the resolution of the cryoEM maps, so channel opening does not seem to induce major conformational rearrangements within each hot spot. Full size image The study by Samso et al. [14] is the only one that systematically compared the open and closed states at a resolution ~10 Å. Comparing the docking in two other cryoEM maps near ~10 Å [15] , [30] also supports the idea that channel opening coincides with a widening of the intersubunit gap ( Supplementary Fig. S2 ). Many mutations were previously found at interfaces involving domains A, B and C within a single subunit [16] . Could these interfaces also be disrupted as part of channel opening, and could those disease mutations therefore also facilitate channel opening? A direct superposition of domain A of the open- and closed-state models shows that the intrasubunit domain–domain movements would be more subtle ( Fig. 2b ), with shifts of domains B and C relative to domain A of ~2–3 Å, which are too small to be interpreted at the given resolution of the cryoEM maps. Because there do not seem to be major relative movements at the intrasubunit interfaces upon opening, we decided to further investigate disease-associated mutations at the various intrasubunit interfaces between domains A, B and C. Disease mutations can weaken the thermal stability MH is the result of increased sensitivity of RyR1 to halogenated anaesthetics. In addition, many mutations in RyR1 have also been associated with increased temperature sensitivity, and may underlie environmental heat stroke [31] , [32] , [33] , [34] , [35] , [36] , [37] , [38] . We prepared nine different disease-associated mutants of RyR1ABC, all of which are associated with a gain-of-function phenotype ( Supplementary Table S1 ). They are located at the interfaces between domains A, B and C, or are buried within individual domains ( Fig. 3a ). Other RyR1 mutations located at the periphery of the hot spot were not included, as their effect would only become clear in the presence of neighbouring domains. Thermal stability measurements show that wild-type RyR1ABC has a melting temperature of ~47 °C, and several (but not all) mutations lowered the thermal stability, with a maximum effect of >9 °C destabilization for the C36R mutant ( Fig. 3b , Supplementary Fig. S3 ). The lowered stability of some RyR1 mutations may directly underlie a temperature-sensitive phenotype. For example, the R402C mutation (rabbit RyR1 numbering), which is similar to the R402G mutation that destabilizes the hot spot by >5 °C, has been associated with rhabdomyolysis triggered by exercise in hot weather [39] . 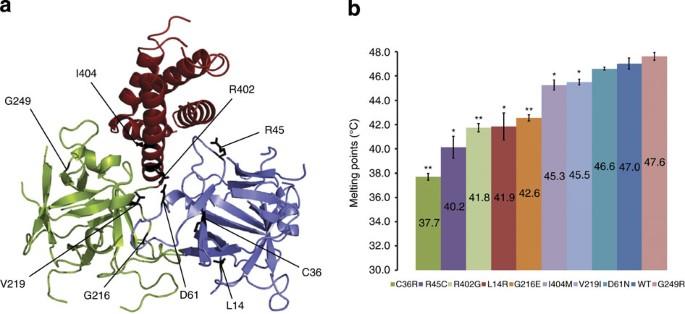Figure 3: Thermal melt analysis. (a) Overview of the positions of nine different mutations included in the thermal melt study. (b) Average melting temperatures of wild-type RyR1ABC and nine different disease mutants using thermofluor experiments (n=4 for each). The error bar indicates the s.d. (statistical analysis was performed using two-tailed, paired Student’st-test). *P<0.02 and**P<0.001. The actualP-values are (for comparison with wild type): C36R (3.3 × 10−5), R45C (0.0016), R402G (8.2 × 10−4), L14R (0.0029), G216E (6.2 × 10−4), I404M (0.0073), V219I (0.019), D61N (0.20) and G249R (0.17). Figure 3: Thermal melt analysis. ( a ) Overview of the positions of nine different mutations included in the thermal melt study. ( b ) Average melting temperatures of wild-type RyR1ABC and nine different disease mutants using thermofluor experiments ( n =4 for each). The error bar indicates the s.d. (statistical analysis was performed using two-tailed, paired Student’s t -test). * P <0.02 and ** P <0.001. The actual P -values are (for comparison with wild type): C36R (3.3 × 10 −5 ), R45C (0.0016), R402G (8.2 × 10 −4 ), L14R (0.0029), G216E (6.2 × 10 −4 ), I404M (0.0073), V219I (0.019), D61N (0.20) and G249R (0.17). Full size image Buried disease mutations affect the intersubunit interface A small number of disease mutations are buried within individual domains. We analysed the effect of three such mutations (L14R, G216E and G249R) on the structure of the N-terminal disease hot spot. The G216E mutant expressed well with an intermediate destabilization ( Fig. 3b ), but did not crystallize. The G216 C α atom is buried within domain B, and an E216 side chain would clash with a neighbouring β strand (β16). The inability to crystallize suggests that the structural changes are quite substantial. However, as circular dichroism (CD) spectra of wild type and mutant are nearly identical ( Supplementary Fig. S4 ), the changes do not seem to involve secondary structure content, and may include relative domain movements or increased flexibility. The G249R mutant introduces a bulky Arg side chain within a buried region of domain B ( Fig. 4a , Supplementary Fig. S5a ). Its thermal stability is not altered significantly ( Fig. 3b ), but the mutant displaces the neighbouring side chains of E229 and L372. In addition, the neighbouring loop 226–229 ( Fig. 4a , red), which is partially disordered in the wild-type structure, has an altered conformation and is now completely visible. This loop harbours the positions of four different disease mutations (including E229) in RyR1 and RyR2 combined and is located at the intersubunit interface 1 between two neighbouring ABC structures. 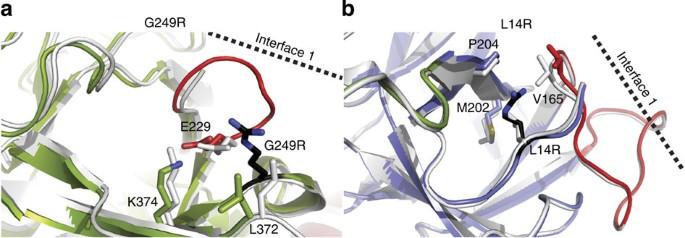Figure 4: Buried disease mutations. Superposition of the wild-type (white) and mutant (colours) structures for (a). G249R (Protein Data Bank (PDB) ID: 4I1E) and (b). L14R (PDB ID: 4I7I). Blue: domain A. Green: domain B. The mutated residue is shown in black. Loops directly located at interface 1 are shown in red. Figure 4: Buried disease mutations. Superposition of the wild-type (white) and mutant (colours) structures for ( a ). G249R (Protein Data Bank (PDB) ID: 4I1E) and ( b ). L14R (PDB ID: 4I7I). Blue: domain A. Green: domain B. The mutated residue is shown in black. Loops directly located at interface 1 are shown in red. Full size image L14R introduces a charged residue in a small hydrophobic core near the very amino terminus, including V165, M202 and P204 ( Fig. 4b , Supplementary Fig. 5b ). The mutation displaces the main chain and side chain of V165, which is located on the β8-β9 loop of domain A, also located at interface 1. Although L14R and G249R represent buried mutations, they both seem to affect an interface that is altered upon channel opening. Salt-bridge mutations cause relative domain–domain movements Three RyR1 mutants (R45C, D61N and R402G) target ionic pairs between domains A and C. They cause the largest structural changes, evoking relative domain–domain movements. R45C breaks a salt bridge with D447 on domain C. This causes the D447 side chain to become unstructured, and domain C to pivot with displacements up to ~3 Å near the cytoplasmic side of the helical bundle ( Fig. 5a ; Supplementary Movie 3, Supplementary Fig. S5c ). 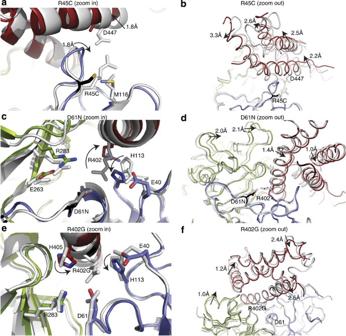Figure 5: Disease mutations affecting interdomain ionic pairs. (a,b). R45C (Protein Data Bank (PDB) ID: 4I6I). (c,d) D61N (PDB ID: 4I3N). (e,f) R402G (PDB ID: 4I37). All superpositions are based on domain A. Colour scheme as inFig. 4. Arrows indicate changes relative to the wild-type structure. R45C and R402G are in comparison with the wild-type structure crystallized in PA5100. Figure 5: Disease mutations affecting interdomain ionic pairs. ( a , b ). R45C (Protein Data Bank (PDB) ID: 4I6I). ( c , d ) D61N (PDB ID: 4I3N). ( e , f ) R402G (PDB ID: 4I37). All superpositions are based on domain A. Colour scheme as in Fig. 4 . Arrows indicate changes relative to the wild-type structure. R45C and R402G are in comparison with the wild-type structure crystallized in PA5100. Full size image Both D61 and R402 are involved in a salt bridge, together with E40. The D61N mutation is isosteric, neutralizing a negative charge ( Fig. 5c , Supplementary Fig. S5d ). This causes a complete disruption of the ionic pair network, with R402 swinging away, breaking the interactions with both N61 and E40, and causing a relative change in the orientation of domain C with displacements close to 1 Å. In domain B, R283 is no longer attracted to the negatively charged D61, causing a relative reorientation of domain B with shifts ~2 Å ( Fig. 5d ). The R402G mutation disrupts the same ionic pair network. H113 and H405 close the gap created by taking away the long Arg side chain ( Fig. 5e , Supplementary Fig. S5e ), and the domain C backbone has shifted by up to ~2.5 Å relative to domain A ( Fig. 5f ). Although domains A, B and C interact through multiple ionic pairs, disruption of even single ones is sufficient to cause relative domain reorientations. This shows how mutations located at the interfaces between domains A, B and C can affect regions at the periphery of the hot spot. Keeping domain C fixed, for example, the mutations would affect the positions of domain A and B, and hence, again, the intersubunit interface 1. Uncharged mutations at the A–B–C interface cause local changes We looked at the effect of three additional mutants at the intrasubunit interfaces between domains A, B and C that do not disrupt ionic pairs (C36R, V219I and I404M). The C36R mutant caused the largest effect on the melting temperature ( Fig. 3b ). C36 is located at the surface of domain A, and has only minor effects on the structure of domain A in isolation [18] . However, it is buried at the interface between domains A and B, and a direct placement of an Arg residue would clash with domain B. The mutation has several profound effects on the structure ( Supplementary Movie 4 ). First, a neighbouring loop in domain A (residues 52–60) moves ~2 Å to allow the R36 side chain to fit in a folded, rather than an extended, conformation ( Fig. 6a , Supplementary Fig. S5f ). This prevents a direct clash with domain B, but the moving loop contains several contact points with domain B in the wild-type structure, and thus affects the domain A–B interface. The Q23 and N203 side chains move towards the R36. The altered N203 side-chain conformation, together with the longer R36 side chain, cause the neighbouring domain B loop to be displaced by ~1 Å. All together, these significantly affect the A–B interface, destabilizing the RyR1ABC protein by ~9 °C ( Fig. 3b ). 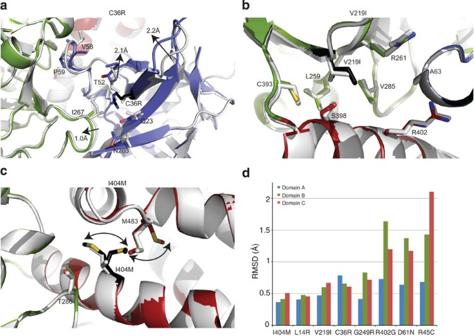Figure 6: Other mutations at the intrasubunit interfaces between different domains. (a) C36R (Protein Data Bank (PDB) ID: 4I0Y). (b) V219I (PDB ID: 4I8M). (c) I404M (PDB ID: 4I2S). Colour scheme as inFig. 4. For I404M, dual conformations were observed in the electron density. Arrows indicate changes relative to the wild-type structure. (d) RMSD values for superposition of the mutants with the wild-type structure. The superposition is performed based on domain A, so the values for domains B and C are the sum of intrinsic structural differences within the domains and relative domain reorientations compared with the wild-type structure. R402G and R45C are in comparison with the wild-type structure crystallized in PA5100. Figure 6: Other mutations at the intrasubunit interfaces between different domains. ( a ) C36R (Protein Data Bank (PDB) ID: 4I0Y). ( b ) V219I (PDB ID: 4I8M). ( c ) I404M (PDB ID: 4I2S). Colour scheme as in Fig. 4 . For I404M, dual conformations were observed in the electron density. Arrows indicate changes relative to the wild-type structure. ( d ) RMSD values for superposition of the mutants with the wild-type structure. The superposition is performed based on domain A, so the values for domains B and C are the sum of intrinsic structural differences within the domains and relative domain reorientations compared with the wild-type structure. R402G and R45C are in comparison with the wild-type structure crystallized in PA5100. Full size image The V219I mutation is located at the B–C interface and is very subtle, as it only introduces a single methyl group. It is surrounded by mostly hydrophobic residues, but no appreciable effect is seen on the structure ( Fig. 6b , Supplementary Fig. S5g ). The only effect could be that the hydrophobic packing is less-than-ideal, but as expected, the effect on the thermal melting is also minimal ( Fig. 3b ). The I404M mutation is near the B–C interface. Interestingly, this mutation causes a clash with M483 in domain C. As a result, both M404 and M483 adopt dual conformations ( Fig. 6c , Supplementary Fig. S5h ). The branched C γ atom of I404 is in Van der Waals contact with T286 on domain B in the wild-type structure. These changes result in a relatively small drop (~2 °C) in melting temperature ( Fig. 3b ). Figure 6d shows the root mean square deviation (RMSD) values for each domain, after superposing the modelled C α atoms in domain A. The values for domains B and C thus also indicate their degree of movement relative to domain A. Overall, the V219I and I404M mutants are predicted to have the smallest functional impact, as these mutants do not cause large structural changes and have only modest effects on the melting temperatures. Most mutants crystallized in the same condition reported for WT RyR1ABC, but two of them, R45C and R402G, crystallized in different conditions involving a polyacrylic acid (PA5100). We also crystallized the wild-type protein in PA5100, which was at lower resolution (3.5 Å) but allowed us to investigate the relative domain orientations. The RMSD values and figures for R45C and R402G superpositions are based on comparison with WT protein in PA5100, showing that the conformational changes are due to the mutations, and not the crystallization conditions. None of the observed conformational differences are due to pH changes ( Supplementary Fig. S6 ). The relative orientation of domains B and C As breaking favourable interactions between domains A–B or A–C causes relative domain reorientations, we wondered whether the destabilization simply allows a preferred relative orientation between domains B and C. In this scheme, domain A would act as a ‘clamp’ that prevents the most favourable interactions between domains B and C. This situation is then analogous to IP 3 receptors where domain A, also known as the suppressor domain, decreases the ligand-binding affinity by clamping domains B and C in a conformation that disfavours IP 3 binding [23] , [24] , [40] , [41] . We therefore solved the structure of domains B and C in the absence of domain A. Superposition of domain B shows that the relative orientation of domain C differs appreciably between the RyR1ABC and RyR1BC crystal structures ( Supplementary Figs. S5i and S7 ). In the absence of domain A, domain C swings towards the position of domain A, showing that domain A prevents a more favourable interaction between domains B and C through steric hindrance. The results suggest that weakening the A–C interaction through disease mutations allows more favourable B–C interactions to occur. However, the disease mutations cannot cause the exact same B–C reorientation because domain A still provides steric hindrance. RyRs are allosteric membrane proteins, whose major function is to release Ca 2+ from the endoplasmic or sarcoplasmic reticulum. Primary triggers for channel opening include cytoplasmic and luminal Ca 2+ , as well as voltage-dependent conformational changes in the L-type calcium channel Ca V 1.1. These likely cause channel opening by stabilizing open-state or destabilizing closed-state conformations of the cytoplasmic portion. Disease-causing mutations in RyR1 and RyR2 interfere with channel gating. With some exceptions, most mutants have been associated with a gain-of-function, for example, by lowering the threshold for activating ligands. Several theories have been put forward to explain their effect. In the ‘zipper hypothesis’, it was postulated that the N-terminal and central disease hot spots interact, and that disease mutations are located at their interface [42] . However, it is now clear that most disease mutations in the N-terminal region are already involved with other domain–domain interfaces, and only a small fraction could remain available for binding the central hot spot [16] . It was also postulated that the mutations may affect the binding of FK506-binding proteins (FKBPs), and that the resultant dissociation facilitates channel opening [43] , [44] , [45] , [46] . One group suggested that the N-terminal region might interact directly with FKBPs [47] , but our isothermal titration calorimetry (ITC) experiments failed to detect any appreciable binding ( Supplementary Fig. S8a ). This is in agreement with cryoEM studies showing that FKBPs bind at the periphery of the cytoplasmic foot (for example, see Samso et al. [48] ), far away from the docked position of the N-terminal disease hot spot. Here we built pseudo-atomic models of the N-terminal region in the open and closed states of RyR1, which suggest that channel opening results in ~7 Å widening of an intersubunit contact area. One likely interpretation is that there are direct contacts between domains A and B of neighbouring subunits in the closed state, and that those contacts are disrupted or drastically altered as the channel opens. The interaction thus serves as a ‘brake’ on channel opening, imposing an energetic barrier that needs to be overcome to allow channel opening ( Fig. 7 ). This energy would be delivered by binding of triggering agents like Ca 2+ , which likely cause long-range conformational changes that couple allosterically to the N-terminal region. This also implies that the contacts must be extremely weak: a high-affinity interaction would require an extremely high energetic penalty for disruption, as the effective concentration of two juxtaposed segments within a macromolecule can be in the molar range [49] . Indeed, using various approaches (pull-down experiments, cross-linking, gel filtration chromatography and ITC), we failed to observe any interactions between individual RyR1ABC monomers in solution, implying that they do not drive tetramerization. The latter was shown to be mediated by the C-terminal area, which contains a coiled coil region [50] . The proposed intersubunit interactions in the N-terminal region can therefore only arise in the context of a high effective concentration. The same applies to interactions between domain A and domains B and C within a subunit, as the two separately purified constructs also failed to show any interaction in solution, despite their unambiguous contacts in the crystal structure ( Supplementary Fig. S8b ). 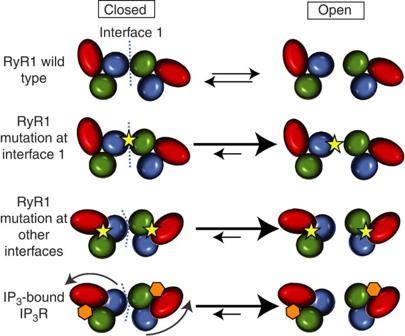Figure 7: Model for the effect of N-terminal disease mutations in RyRs and ligand binding in IP3R. Wild-type RyR1: channel opening requires breaking the interaction along interface 1 between two neighbouring N-terminal disease hot spots. This involves an energetic penalty. Disease mutations directly at interface 1 weaken the interaction, which reduces the energetic penalty and facilitates channel opening. Some disease mutations within a hot spot can change the relative domain–domain orientations, thus affecting other interfaces at the periphery of the hot spot, such as interface 1. These long-range structural changes therefore also facilitate channel opening. In IP3R, binding of IP3(hexagon) results in relative domain reorientations, which also affects interface 1 and facilitates channel opening. Figure 7: Model for the effect of N-terminal disease mutations in RyRs and ligand binding in IP 3 R. Wild-type RyR1: channel opening requires breaking the interaction along interface 1 between two neighbouring N-terminal disease hot spots. This involves an energetic penalty. Disease mutations directly at interface 1 weaken the interaction, which reduces the energetic penalty and facilitates channel opening. Some disease mutations within a hot spot can change the relative domain–domain orientations, thus affecting other interfaces at the periphery of the hot spot, such as interface 1. These long-range structural changes therefore also facilitate channel opening. In IP 3 R, binding of IP 3 (hexagon) results in relative domain reorientations, which also affects interface 1 and facilitates channel opening. Full size image Incidentally, the intersubunit contact area between domains A and B contains the largest cluster of disease mutations within the N-terminal region (20 for RyR1 and RyR2 combined) ( Fig. 2a ), all of which are associated with gain-of-function phenotypes (MH and catecholaminergic polymorphic ventricular tachycardia) [16] . How could these affect channel opening? Mutations in the domain A β8-β9 loop, one of the loops located at the contact region, were previously found not to cause any structural or stability differences [17] , [18] . This implies that their only possible involvement is to be located at a functional interface, and we propose that they form part of intersubunit interactions that are disrupted upon channel opening. When a random disease mutation is introduced, there is a much higher probability that the mutation will weaken, rather than strengthen the intersubunit contacts. Such mutations will lower the energy barrier to open the channel, which in turn facilitates channel opening ( Fig. 7 ). Important to point out is that they do not cause channel opening themselves. They simply weaken the ‘brake’ on channel opening, and some amount of energy, albeit less, is still needed through binding of triggering agents. This can, for example, explain the shift in Ca 2+ dependence and voltage dependence of channel opening [51] , [52] . Many mutations are not located at the intersubunit interface. However, we previously observed that most mutations in the N-terminal disease hot spot are located at domain–domain interfaces, including the interfaces between domains A, B and C within individual subunits [16] . We found that several mutations that disrupt salt bridges between domains A and C can cause relative domain movements. Therefore, such mutations cause long-range structural changes, which automatically affect the interfaces at the periphery of these domains. One straightforward interpretation is that this domain ‘misalignment’ also affects the intersubunit interface 1, and thus also lowers the energetic barrier to open the channel ( Fig. 7 ). In full-length RyRs, the relative domain orientation could be stabilized by surrounding domains. However, even if the ABC domains have the wild-type orientation in full-length RyR mutants, there is now additional strain on the other interfaces to keep the ABC domains positioned. For example, if the interactions across interface 1 can keep the mutant ABC domains in a wild-type orientation, away from their favoured orientation in isolation, then this reduces the stability of the closed state. Upon channel opening, the mutant ABC domains can then relax back to their favoured orientation. The closed state is thus destabilized relative to the open state, resulting in facilitated channel opening. Mutations that are buried (G249R and L14R) also seem to affect the intersubunit interface through conformational changes that couple within the protein. These results highlight the overall importance of this interface in channel opening. Finally, some mutations did not seem to cause any large structural changes, but only had an effect on the thermal stability (V219I and I404M). The largest effect was observed for the C36R mutation, destabilizing the RyR1ABC protein by >9 °C ( Fig. 3b ). The altered melting temperatures imply that there may be temperature-dependent conformational changes, which could then also affect one or more individual domain interactions. The RyR N-terminal region shares ~21% sequence identity with the corresponding region in IP 3 Rs, suggesting that both channels may have adopted similar allosteric strategies [41] . In IP 3 Rs, the N-terminal domain A is also known as the ‘suppressor’ domain, which lowers the affinity for IP 3 by clamping domains B and C in a conformation that is unfavourable for IP 3 binding [40] . Importantly, domain–domain reorientations have also been observed in IP 3 RABC through binding of IP 3 (refs 23 , 24 ), suggesting a common theme in both types of calcium-release channels ( Fig. 7 ). In RyRs, the relative domain orientation can be altered permanently through a disease mutation, whereas in IP 3 Rs, the reorientation is reversible through binding and unbinding of IP 3 (refs 23 , 24 ). The IP 3 RABC domains also dock near the four-fold symmetry axis of a 9.5 Å IP 3 R cryo-EM map [53] , making intersubunit contacts that are very similar to the RyR1ABC interactions [23] . It has been suggested before that IP 3 binding may also rearrange the intersubunit interface [23] . Future cryoEM studies comparing open and closed IP 3 Rs may show a similar widening of the intersubunit gaps. Whether an activator can bind the RyR N-terminal region and cause domain rearrangements similar to IP 3 in IP 3 Rs remains to be discovered. Throughout the manuscript, all numbering corresponds to the amino-acid sequence of rabbit RyR1. CryoEM docking The RyR1ABC crystal structure (Protein Data Bank: 2XOA) was docked into open and closed RyR1 cryoEM reconstructions described by Samso et al. [14] (Electron Microscopy Data Bank (EMDB) accession codes 1607 and 1606, respectively). The full structure was placed four times in the four-fold symmetric map using extensive six-dimensional searches using the colores program in the Situs 2.6 package [55] . Contrast plots, showing the correlation coefficients of the top solutions, were prepared based on this docking. The positions of all twelve individual domains were further refined by rigid-body refinement, taking steric clashes into account as implemented in the collage program of Situs 2.6 (ref. 55 ). A Laplacian filter was applied during all stages. The pseudo-atomic models are available as Supplementary Data 1 (closed, EMDB: 1606) and Supplementary Data 2 (open, EMDB: 1607). Cloning and crystallization of disease mutants RyR1ABC proteins (wild type and mutants) were expressed and purified as described previously [16] , with the difference that most constructs encompassed residues 1–536 instead of 1–559, because the C-terminal 27 residues were found to be unstructured. The exception is the R45C mutant, where the 1–559 construct was used for crystallization. All thermal melts were performed on the 1–536 constructs. The RyR1BC construct (residue 217–536) was cloned in the same pET28HMT vector as described before [16] and purified using a similar strategy as for RyR1ABC, with the following differences. After cleavage with Tobacco Etch Virus (TEV) protease and collecting the PorosMC flowthrough, the sample was run on a ResourceQ column (GE Healthcare) in 20 mM Tris-Cl pH 8.0, 14 mM β-mercaptoethanol (β-ME), with a gradient from 50 to 350 mM KCl, and on a Phenyl Sepharose column (GE Healthcare) in 20 mM Tris-Cl pH 8.0, 14 mM β-ME, with a gradient from 50–1500, mM KCl. The sample was then run on a preparative Superdex 200 as for the RyR1ABC proteins. Before crystallization, the proteins were exchanged to 50 mM KCl, 10 mM Na-Hepes pH 7.4, 10 mM dithiothreitol (DTT) and concentrated to 10 mg ml −1 using a 10,000 MWCO concentrator (Amicon, Millipore). All crystals were obtained using the hanging drop method at 4 °C. L14R and D61N were crystallized in 1.4–1.6 M ammonium sulphate (AS) and 0.1 M HEPES pH 8.0 or 0.1 M Bicine pH 9.5, respectively. V219I was crystallized in 1.4 M AS, 12% glycerol and 0.1 M Bicine pH 9.0. G249R and I404M were crystallized in 1.3–1.5 M AS, 12% glycerol and 0.1 M Tris pH 8.0. To verify the impact of pH on the structure, we also crystallized wild-type RyR1ABC in AS at three different pH values (pH 8.0, 9.0 and 9.5). C36R was crystallized in 1.2 M lithium sulphate and 0.1 M Bicine pH 9.5. R45C and R402G were crystallized in 20–22% PA5100 sodium salt (PA5100), 0.02 M MgCl 2 and 0.1 M HEPES pH 7.0 or 0.1 M Bis-Tris pH 6.5, respectively. RyR1BC crystals were obtained in 0.1 M Tris-Cl pH 7–8, 100–250 mM KCl and 20–30% PEG 3350. All crystals were flash frozen in the corresponding mother liquor containing 25–30% glycerol. Data collection and refinement Data were collected at beamline 9-2 of the Stanford Synchrotron Radiation Laboratoray (Menlo Park) and 08ID of the Canadian Light Source (Saskatoon). The data were processed using the HKL2000 package (HKL Research) and XDS [56] . All structures were solved using molecular replacement implemented in Phaser [57] , using individual domains as search models. Refinement consisted of successive rounds of manual modelling in COOT [58] and refinement in REFMAC5 [59] with TLS restraints applied to individual domains. Data collection and refinement statistics are available in Table 1 . Coordinates and structure factors for all described structures are available in the Protein Data Bank (to be deposited and will be available upon publication). Superpositions and RMSD calculations were performed using ProFit ( http://www.bioinf.org.uk/software/profit ). The structures of wild-type RyR1ABC at pH 8, 9 and 9.5 were identical, indicating that the observed structural differences for the mutations were not due to differences in pH ( Supplementary Fig. S6 ). Table 1 Crystallographic parameters Full size table Thermal melt analysis The protein melting curves were measured by means of thermofluor experiments [60] . Samples for melting curves contained 50 μl of 0.2 mg ml −1 protein and 1 × SYPRO Orange solution (Invitrogen) using the manufacturer’s instructions. The melts were obtained in a DNA engine opticon 2 real-time PCR machine (Bio-Rad), using the SYBR green filter option. The temperature was changed from 20 to 95 °C in 0.5 °C steps. At every step, the temperature was kept constant for 15 s. The melting temperatures were obtained by taking the midpoint of each transition. CD spectra measurement CD spectra of RyR1ABC WT and G216E were measured in buffer containing 50 mM KCl and 10 mM Na 3 PO 4 (pH 7.4). Concentrations were determined using the calculated extinction coefficient at 280 nm in the presence of 6 M guanidine. CD spectrum measurements were performed using a Jasco J810 CD spectropolarimeter on samples at a concentration of 2 μM. CD spectra of the samples and buffer alone were collected over a spectral window of 195–280 nm at 22 °C. Isothermal titration calorimetry experiments A clone for GST-FKBP12 was obtained from Dr Wayne Chen (University of Calgary), and expressed in Escherichia coli Rosetta (DE3) pLacI at 37 °C, induced at an OD 600 of ~0.6 by addition of 0.2 mM isopropyl-β- D -thiogalactoside for 4 h. Cells were lysed by sonication in buffer A (250 mM KCl, 10 mM β-ME and 10 mM HEPES, pH 7.4), with 25 mg ml −1 DNase I, 25 mg ml −1 lysozyme and 1 mM phenylmethylsulphonyl fluoride. The lysate was loaded on to a GSTPrep FF 16/10 column (GE Healthcare) equilibrated with buffer A. The column was washed with three column volumes (CVs) buffer A and eluted with two CV buffer B (buffer A+10 mM reduced glutathione). The eluate was dialyzed against buffer C (10 mM KCl, 20 mM TRIS, pH 8.0). The dialyzed protein was applied to a HiLoad 16/10 Q-Sepharose HP column (GE Healthcare) equilibrated with buffer C. The protein was eluted with a gradient of 0–50% buffer D (1.5 M KCl, 20 mM TRIS, pH 8.0) over 18 CV. Fractions containing protein were concentrated and applied to a Superdex 75 10/300GL column (GE Healthcare). The correct molecular weights for both proteins was confirmed by MALDI-TOF on a Voyager-DE STR (Applied Biosystems). Before ITC experiments, GST-FKBP12 and wild-type RyR1ABC were dialyzed overnight against 150 mM KCl, 10 mM HEPES, pH 7.4 and 10 mM β-ME at 4 °C. Concentrations were determined using the calculated extinction coefficient at 280 nm in the presence of 6 M guanidine. GST-FKBP12 (1.627 mM) was used as titrant, and 20 injections of 2 μl each were titrated into RyR1ABC at 10-fold lower concentration. The data were processed using Origin 7.0. Accession codes: The RyR N-terminal mutant and domain BC structures generated in this study have been deposited in the Protein Data Bank under the following accession codes: 4I96 ( Supplementary Figs S5 and S7 ), 4I8M, 4I7I, 4I6I, 4I3N, 4I37, 4I2S, 4I1E and 4I0Y. How to cite this article: Kimlicka, L. et al. Disease mutations in the ryanodine receptor N-terminal region couple to a mobile intersubunit interface. Nat. Commun. 4:1506 doi: 10.1038/ncomms2501 (2013).